Whole-exome sequencing implicates UBE3D in age-related macular degeneration in East Asian populations Age-related macular degeneration (AMD) is a leading cause of irreversible central blindness among the elderly worldwide. We use exome sequencing to analyse nonsynonymous single-nucleotide variants (SNVs) across the whole genome of 216 neovascular AMD cases and 1,553 controls. As a follow-up validation, we evaluate 3,772 neovascular AMD cases and 6,942 controls from five independent cohorts in the East Asian population. Here we show strong evidence of an association at a novel, missense SNV, rs7739323, which is located in the ubiquitin protein ligase E3D ( UBE3D ) gene ( P meta =1.46 × 10 −9 , odds ratio (OR)=0.74, 95% confidence interval (CI): 0.63–0.88). Furthermore, ablation of the UBE3D protein lead to an abnormal amount of pigment granules deposited in retinal pigment epithelium microvilli area and an abnormal response on electroretinography (ERG) in UBE3D +/− heterozygous mice. Our findings indicate that the ubiquitin-proteasome system may play a role in the pathogenesis of neovascular AMD. Age-related macular degeneration (AMD) is a leading cause of irreversible central blindness among the elderly worldwide [1] . Neovascular AMD is a subtype of advanced AMD and is responsible for >80% of severe vision loss caused by AMD [2] . The aetiology of AMD is multifactorial and is affected by age, the environment, and genetic susceptibility [3] , [4] , [5] . Previous genome-wide association studies have identified numerous risk-associated variants within 19 susceptibility loci for AMD [6] , [7] , [8] , [9] , [10] . However, genome-wide association studies focus on common variants (minor allele frequency (MAF) >5%), which are usually located in the intronic regions of the chromosome and do not encode specific functional proteins [11] , [12] . The functional coding variants in these susceptibility loci have not been systematically investigated. Whole-exome sequencing (WES)-based studies are emerging as a popular approach to test for the association of coding variants with complex traits and diseases [13] , [14] , [15] . Exome sequencing evaluates the exonic regions of the chromosome, which constitute ∼ 1% of the entire genome and encode functional proteins. It is possible to obtain deep coverage, which is necessary for the detection of variants, with relatively few reads [16] . Therefore, there is strong interest in exome sequencing because of its potential to identify genes underlying complex traits and enable straightforward functional annotation of coding variation [15] . The purpose of the present study is to identify the genetic variants that confer susceptibility to neovascular AMD. We screen the susceptibility loci for neovascular AMD in the coding exome using WES. Then, we validate the contribution of functional coding variants to genetic susceptibility for AMD in six independent samples. Furthermore, we generate UBE3D +/− heterozygous mice (no UBE3D −/− mice survives) and perform electron microscopy to investigate the structural changes and electroretinography (ERG) to measure retina function. Our findings indicate that the ubiquitin proteasome system (UPS) may play a role in the pathogenesis of neovascular AMD. 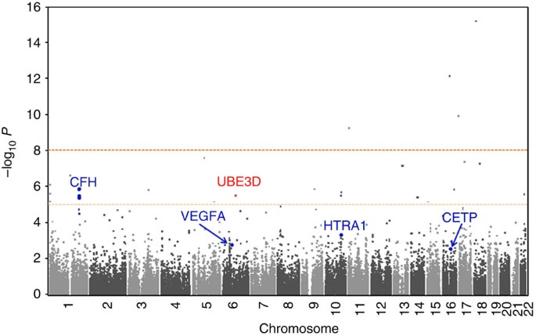Figure 1: Manhattan plot for exome sequencing. The association results of the single-variant analysis (χ2-test is used for association testPvalue (−log10P); 216 neovascular AMD cases and 1,553 controls are used) are plotted against the genomic position. The previously identified loci are presented in blue, and the locus that was identified in the current study is presented in red. SNP associations in the exome-sequencing discovery cohort In the discovery stage, we performed WES of 216 neovascular AMD cases and 1,553 controls ( Table 1 , Supplementary Fig. 1 and Supplementary Table 1 ) with sequence coverage of ∼ 31X, and we identified 62,870 single-nucleotide polymorphisms (SNPs). Overall genomic inflation was very low ( λ gc=1.02; Supplementary Fig. 2 ), suggesting minimal confounding of the disease association analysis by population stratification or other systematic study design biases. 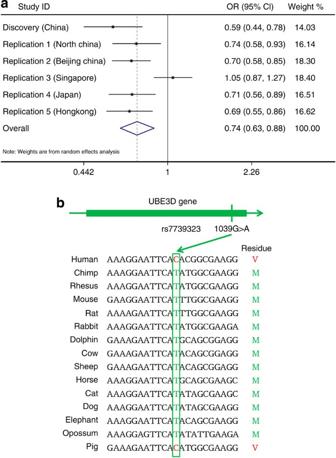Figure 2: OR plot and homolog study of rs7739323. (a) The OR plot shows the allelic effects of the T allele of rs7739323 in the discovery stage (216 AMD cases and 1,553 controls) and in the 5 independent cohorts (803 AMD cases and 395 controls of North China, 850 AMD cases and 856 controls of Beijing China, 507 AMD cases and 2,967 controls of Singapore, 981 AMD cases and 757 controls of Japan, 631 AMD cases and 1,967 controls of Hong Kong).Pvalues were generated using logistic regression under the additive model and are presented in parentheses. The error bars represent the 95% confidence intervals (CIs) of the ORs. (b) The homolog study showed that theUBE3Dgene is conserved in most animals. However, most animals have a T at this position, whereas only humans and pigs have a C at this position. Of these variants, 27.08% were nonsynonymous ( Supplementary Table 2 and Supplementary Fig. 2 ). We identified 40,062 SNPs that were previously reported in the Single Nucleotide Polymorphism Database (dbSNP) and 22,808 novel SNPs ( Fig. 1 ). 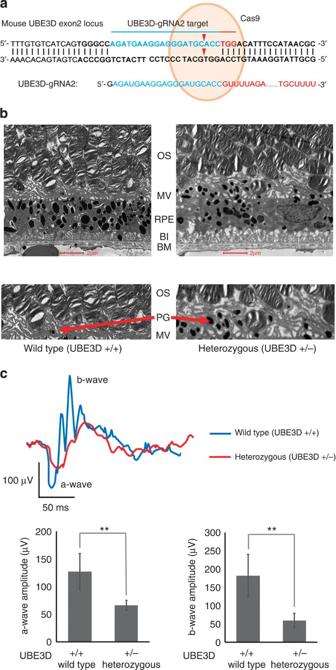Figure 3: Generation and characterization of heterozygousUBE3D+/−mice. (a) Schematic representation of theUBE3Dgene knockout strategy in mice (we obtainedUBE3D+/−heterozygous mice, noUBE3D−/−mice survived). (b) Electron microscopy showed more loose retinal pigment epithelium microvilli and more pigment granules (PG) in 3-month-oldUBE3D+/−heterozygous mice than in wild-type mice. Scale bars, 2 μm. (c) ERG demonstrated a lower a-amplitude and b-amplitudein 3-month-old heterozygousUBE3D+/−mice than in age-matched controls.N=6. BI, basal infolding; BM, Bruch's membrane; OS, outer segment of receptor cells; MV, microvilli. The bar in the graph represents the s.e.m. Student’st-test, **P<0.001. Compared with the SNPs in the 1000 Genomes Project (China Han+Japan Tokyo (CHB+JPT), 2010, 3), the recovery rate of common SNPs (MAF≥5%) was 91.4% ( Supplementary Table 3 ), suggesting a low false-negative rate in our data. In addition, we performed a validation assay using mass spectrum genotyping technology on 79 randomly selected SNPs in 252 exome-sequenced samples ( Supplementary Table 4 ). The genotype concordance rate between the genotyping and sequencing was 99.5% (19281/19387), demonstrating the high quality of our sequencing data and the accuracy of our genotype calling. Initial association analyses performed using the 216 AMD cases and 1,556 controls from this discovery stage confirmed previously reported associations of AMD with sequence variants mapping to CFH , HTRA1 , B3GALTL , C2 and SKIV2L ( Supplementary Table 5 ). UBE3D is not a highly polymorphic gene in the East Asian population. The MAF of rs7739323 is between 0.13 and 0.15 in the Chinese population, and 0.09 in the Japanese (according to the 1000 Genomes project; http://www.1000genomes.org/ ). In our study, the MAF ranged from 0.13 to 0.22 in the control Chinese population and was 0.11 in the Japanese population ( Supplementary Fig. 3 ). The transition/transversion ratio was 2.72 when MAF=0.1–0.2 ( Supplementary Table 6 ). Table 1 Summary of the samples analysed in this study. Full size table Figure 1: Manhattan plot for exome sequencing. The association results of the single-variant analysis ( χ 2 -test is used for association test P value (−log 10 P ); 216 neovascular AMD cases and 1,553 controls are used) are plotted against the genomic position. The previously identified loci are presented in blue, and the locus that was identified in the current study is presented in red. Full size image We performed linkage disequilibrium (LD) analysis of rs7739323 and found that this SNP was not linked with any other previously reported AMD loci in chromosome 6 ( C2-CFB , VEGFA , COL10A1 and IER3-DDR1 ); in addition, no other SNPs were in high LD with rs7739323, which indicates that the results can be attributed to rs7739323 and not neighbouring SNPs ( Supplementary Fig. 4 ). Furthermore, we performed a SKAT-O test, and found that UBE3D was associated with AMD with P =3.55 × 10 −3 , which is consistent with the association of rs7739323 and AMD ( Supplementary Data 1 ). Independent replication of SNP associations and meta-analysis A total of 53 SNP markers not mapping to known AMD loci surpassed P <1 × 10 −4 , and thus were used for replication genotyping in two independent cohorts (North China and Beijing China cohorts), comprising an additional 1,653 cases and 1,251 controls ( Table 2 and Supplementary Table 7 ). We note significant evidence of replication at rs7739323, which encodes a non-synonymous substitution of V>M at position 379 of the gene for UBE3D ( P replication for Northern China =0.011 and P replication for Beijing =2.12 × 10 −4 ; P replication China overall =3.57 × 10 −6 ; Table 2 ). We then evaluated whether this association could be extended outside of China, and thus further assessed it in three additional independent AMD cohorts comprising 2,119 AMD cases and 5,691 controls drawn from Hong Kong, Japan and Singapore. We observed supportive evidence for replication in these three additional samples, yielding a genome-wide significant observation when all six AMD cohorts were meta-analysed ( P meta =1.46 × 10 −9 , odds ratio (OR)=0.78, 95% confidence interval: 0.67–0.90; Fig. 2a ). We note some degree of heterogeneity upon meta-analysis of all six cohorts (heterogeneity χ 2 =16.85, P =0.005, I 2 index=70.3%). However, this heterogeneity arose mainly upon the inclusion of the Singapore cohort. We then repeated the meta-analysis after removing each of the independent cohorts one at a time. No individual study affected the overall OR, as the omission of any single study did not produce a significant difference ( Supplementary Fig. 5 ). Table 2 Results for rs7739323 across cohorts. Full size table Figure 2: OR plot and homolog study of rs7739323. ( a ) The OR plot shows the allelic effects of the T allele of rs7739323 in the discovery stage (216 AMD cases and 1,553 controls) and in the 5 independent cohorts (803 AMD cases and 395 controls of North China, 850 AMD cases and 856 controls of Beijing China, 507 AMD cases and 2,967 controls of Singapore, 981 AMD cases and 757 controls of Japan, 631 AMD cases and 1,967 controls of Hong Kong). P values were generated using logistic regression under the additive model and are presented in parentheses. The error bars represent the 95% confidence intervals (CIs) of the ORs. ( b ) The homolog study showed that the UBE3D gene is conserved in most animals. However, most animals have a T at this position, whereas only humans and pigs have a C at this position. Full size image The homologues study of rs7739323 showed that the UBE3D gene is conserved in most animals. However, most animals have a T at this position. Only humans and pigs have a C at this position ( Fig. 2b ). Generation and characterization of UBE3D +/− heterozygous mice Clustered regularly interspaced short palindromic repeat sequences (CRISPR)-mediated UBE3D knockout mice were generated. However, we did not obtain UBE3D −/− mice. Only heterozygous UBE3D +/− mice survived ( Fig. 3a , and Supplementary Figs 6 and 7 ). Figure 3: Generation and characterization of heterozygous UBE3D +/− mice. ( a ) Schematic representation of the UBE3D gene knockout strategy in mice (we obtained UBE3D +/− heterozygous mice, no UBE3D −/− mice survived). ( b ) Electron microscopy showed more loose retinal pigment epithelium microvilli and more pigment granules (PG) in 3-month-old UBE3D +/− heterozygous mice than in wild-type mice. Scale bars, 2 μm. ( c ) ERG demonstrated a lower a-amplitude and b-amplitudein 3-month-old heterozygous UBE3D +/− mice than in age-matched controls. N =6. BI, basal infolding; BM, Bruch's membrane; OS, outer segment of receptor cells; MV, microvilli. The bar in the graph represents the s.e.m. Student’s t -test, ** P <0.001. Full size image Electron microscopy was performed to evaluate the retinal anatomy of the mice, and it showed more loose retinal pigment epithelium microvilli and more pigment granules (PG) in UBE3D +/− heterozygous mice (3 months old) when compared with age-matched controls ( Fig. 3b ). In ERG, an objective assessment of retinal function, the amplitude of the a-wave and b-wave was decreased in UBE3D +/− heterozygous mice ( Fig. 3c ). These data demonstrate that ablation of the UBE3D protein leads to structural and functional changes in mice. In this study, we performed a comprehensive association analysis on 3,988 neovascular AMD cases and 8,495 controls from East Asia cohorts, and identified a nonsynonymous amino-acid substitution, rs7739323 (encoding for a V>M at position 379 in UBE3D ), that was significantly associated with AMD risk. UBE3D , also known as ubiquitin-conjugating enzyme E2C-binding protein ( UBE2CBP ), accepts ubiquitin from specific E2 ubiquitin-conjugating enzymes and transfers it to substrates, generally promoting their degradation by the proteasome. Moreover, ablation of the UBE3D protein leads to retinal structural changes and abnormal ERG in UBE3D +/− heterozygous mice. Therefore, this study demonstrates a potential link between AMD and the UPS [17] . The cellular ubiquitin–proteasome system, which is important for regulating the intracellular sorting and degradation of proteins, plays a central role in cellular protein homeostasis [17] , [18] . The ubiquitin-conjugating system requires three enzymes: E1, an ubiquitin-activating enzyme; E2, a ubiquitin-conjugating enzyme; and E3, a ubiquitin ligase [19] , [20] , [21] . The ubiquitin ligase recognizes the target protein that is to be degraded. Thus, an association between AMD and the UPS is biologically possible. The retina is an integral part of the central nervous system and, similar to other regions of the brain, it is derived from the neural tube, a precursor of the central nervous system. Consequently, AMD is a neurodegenerative disease [22] , [23] . In the nervous system, the UPS plays a role in normal physiological functions, and evidence gathered over the past decade also indicates a role for the UPS in neurodegenerative diseases [24] , [25] . A previous study found that deficiency in ubiquitin ligase led to the accumulation of neurofilament light chain and to neurodegeneration [26] . Impairment of the ubiquitin–proteasome pathway can also disrupt signal transduction pathways resulting in inflammation and angiogenesis; both are important features of AMD [27] . Therefore, dysfunction of ubiquitin protein ligase (E3) may lead to the accumulation of extracellular deposits (a component of drusen), degeneration of photoreceptors and the retinal pigment epithelium (RPE), and late-stage AMD. Our targeted gene knockout study confirmed the above hypothesis. First, we did not obtain UBE3D −/− mice. Only heterozygous UBE3D +/− mice survived. This suggests that UBE3D , although rarely studied, may play an important role in the development and growth of mice. Second, more pigment granules were deposited in the retinal pigment epithelium microvilliin UBE3D +/− heterozygous mice than in wild-type mice, as demonstrated by the electron microscopy analysis, which indicates that dysfunction of ubiquitin protein ligase (E3) leads to the accumulation of extracellular deposits. Third, heterozygous UBE3D +/− mice displayed severely decline of ERG responses, which shows that a dysfunction of ubiquitin protein ligase (E3) leads to functional changes in the retina. Our results also suggest that rs7739323 is representative of genetic heterogeneity between East Asian regions (Mainland China, Hong Kong and Japan) and South Asia (Singapore). No heterogeneity was found between the Chinese and Japanese cohorts, which may indicate that the association of AMD with the UBE3D variant is only limited to the East Asian population. In addition, we collected the existing data and analysed the effect of age, sex and smoking, and found no significant statistical difference between them ( Supplementary Table 8 ). In summary, we performed a comprehensive analysis of coding single-nucleotide variants in a large sample and uncovered a strong association between AMD risk and a non-synonymous amino-acid substitution within UBE3D in East Asian populations, thus indicating that the UPS may play a role in the pathogenesis of neovascular AMD. Subjects Six independent study cohorts, totalling 12,483 individuals, were evaluated in this study. The samples in the initial stage (China cohort, exome sequencing) included 216 AMD cases and 1,553 controls ( Table 1 , Supplementary Fig. 1 and Supplementary Table 1 ), and were from the Han Chinese population; the samples were obtained through collaboration with multiple hospitals in China. Furthermore, 3,772 AMD cases and 6,942 controls (North China, Beijing China, Singapore, Japan and Hong Kong Cohorts; Table 1 and Supplementary Table 1 ) were recruited in the replication stage. The subjects received a standard ophthalmic examination, including a visual acuity measurement, slit-lamp biomicroscopy and dilated fundus examination, all of which were performed by a retinal specialist. All of the subjects who were diagnosed with AMD underwent fundus fluorescein angiography, optic coherence tomography and indocyanine green angiography. All of the participants provided written informed consent. The study was approved by the ethics committee of Beijing University People’s Hospital and was conducted according to the Declaration of Helsinki principles. The investigators were not blind to group allocation during the experiment when assessing out comes. AMD grading and definition The diagnosis of exudative AMD was made at each site by retinal physicians according to the standard clinical definition. If retinal photographs were available, AMD was also graded following the Wisconsin Age-Related Maculopathy Grading System [28] , the Age-Related Eye Disease Study criteria [29] or the International Classification [19] . The diagnosis of polypoidal choroidal vasculopathy was based on the indocyanine green angiography results using the Japanese Study Group guidelines [30] . Patients demonstrating a branching vascular network that terminated in aneurismal enlargements, that is, polypoidal lesions, and subjects exhibiting other macular abnormalities, such as pathological myopia, idiopathic choroidal neovascularization, presumed ocular histoplasmosis, angioid streaks or other secondary choroidal neovascularization, were excluded from the study. Unaffected subjects were defined as individuals exhibiting no clinical evidence of early or late AMD in either eye or any other eye disease, with the exception of mild age-related cataracts. Subjects with severe cataracts were excluded from the study. Exome sequencing We sequenced 1,769 whole exomes in the first stage of the project at BGI Shenzhen. The genomic DNA for each individual was hybridized with the NimbleGen 2.1M-probe sequence capture array [31] to enrich for exonic DNA in each library. We performed sequencing using the IlluminaHiSeq 2000 platform for each captured library independently to ensure that each sample had an average coverage of ∼ 31-fold. The raw image files were processed using the Illumina Pipeline (version 1.3.4) for base calling with default parameters, and sequences for each individual were generated as 90-bp reads. Alignment and genotype calling The sequence reads were aligned to the human genome assembly hg18 (GRCh36) using SOAP aligner (v2.21) software ( http://soap.genomics.org.cn ) set to a maximum of three mismatches and the parameter set ‘-a -b -D -o -u -r 1 -s 40 -l 35’. The genotype of each position for every sample in a target region was generated using SOAP snp software ( http://soap.genomics.org.cn/soapsnp.html ) with the parameters ‘-i -d -o -r 0.00005 -e 0.0001 -M -t -u -L -s -2 -T’. The SNP sites with high confidence SNPs (quality ≥20 and depth ≥8X) in at least one individual were selected for further analysis. Quality control of samples and SNPs We performed a principal component analysis to control for population stratification; sites with a call rate (quality ≥20 and depth ≥8) >90% were used (1000 Genomes Project data as a reference, release 2010, 3 pilot1) ( Supplementary Fig. 8 ). Pairwise Identical-By-Descent was used to assess the relationship between individuals. The SNP sites that were used for Identical-By-Descent were as follows: (a) call (quality ≥20 and depth ≥8) rate ≥90%; (b) MAF (PLINK)>0.1; (c) LD (plink) ≤0.5; and (d) control Hardy-Weinberg equilibrium (HWE) (PLINK) >0.0001. The cutoff for PIHAT was <0.2, and no related individuals were identified. SNP quality control The following filter criteria were used to control for SNP quality: (a) the SNP should be located in the target region (NimbleGen 2.1M capture kits) and the ±200-bp flanking region; (b) call rate: 90% of the individuals should exhibit high-quality genotypes (quality ≥20 and depth ≥8X); (c) alternative depth: at least one individual should have >4 reads supporting an alternative allele; (d) control HWE test P value ≥10 −4 ; (e) strand bias: the distribution of the major and minor allele should not enrich on either strand; Fisher’s exact test P value ≥1.0 −7 ; (f) homopolymer run ≤6; and (g) end enrichment: the major and minor alleles should not be enriched at the end of the reads, Fisher’s exact test P value ≥1.0 −7 . The missing SNPs that were located in indels in the ±5-bp region were detected using the 1000 Genomes Project ( http://www.1000genomes.org , release 2012, 10, 16). Replication cohorts We examined the association of the top SNPs from our discovery cohort in two independent case–control cohorts ( Supplementary Fig. 1 ).The most highly associated SNP from the discovery cohort was directly genotyped in six replication cohorts. Generation of CRISPR-mediated UBE3D knockout mice The CRISPR-mediated UBE3D knockout mice were produced by Beijing View Solid Biotechnology, China. The linear plasmid pCAG-T7-Cas9 cut by the NotI restriction enzyme was used as the in vitro transcriptional template. After gel purification, Cas9 mRNA was transcribed with the mMESSAGEmMACHINE T7 Ultra Kit (Life Technologies). UBE3D -gRNA2 templates were amplified based on gRNA scaffold using T7 promoter sequence-conjugated primers: T7-UBE3D-g2-FP and gRNA-RP ( Supplementary Table 9 ). UBE3D -gRNA2 was transcribed with a fast in vitro transcription T7 kit (cat. no. VK010, Beijing View Solid Biotechnology, China) and frozen at −80 °C. Zygotes of C57BL/6 mice ( n =120) were injected with Cas9 mRNA and UBE3D-gRNA2 in M2 media (Millipore) using a FemtoJet micromanipulator (Eppendorf, Germany). After microinjection, zygotes were transferred to pseudopregnant females. All mice were maintained in a specific pathogen-free facility. The tail-derived DNA from 2-week-old newborn mice was genotyped by sequencing the PCR products amplified by the primers: UBE3D-sens and UBE3D-anti ( Supplementary Table 9 ). The mutant mice were mated with wild-type C57BL/6 mice to obtain heterozygous UBE3D +/− mice. Western blotting analysis was performed to confirm the UBE3D expression ( Supplementary Fig. 6E and Supplementary Fig. 7 ). The study was approved by the ethics committee of Beijing university people’s hospital. Electron microscopy Fixed tissues were osmicated for 45–60 min in 0.5–1% OsO 4 in 0.1 M cacodylate buffer, processed in maleate buffer for staining with uranyl acetate and resin-embedded [32] . Ultrathin sections were cut at 90 nm using a Leica ultramicrotome and imaged at 80 KeV using a JEOL JEM 1400 electron microscope. Images were captured using a 16-megapixel GATAN Ultrascan 4000 camera. ERG measurement of retina function Heterozygous UBE3D +/− mice and age-matched wild-type mice were dark-adapted overnight and anaesthetized. The coordination of ERG stimulation and the recording of electrical responses were completed using the Phoenix Micron IV Retinal Imaging Microscope (Phoenix, Pleasanton, CA, USA) according to the manufacturer’s instruction manual [33] . The pupils were dilated and a gold-tipped electrode was placed centrally on the cornea. The Ganzfeld mice default setting was used. Two flashes were delivered with a 15-s interval and five responses were averaged. The amplitude of the a-wave and b-wave was recorded. Meta-analysis A meta-analysis across cohorts was performed as previously reported [34] , [35] . The meta-analysis was performed using Stata/SE version 11.0 (Stata Corp., College Station, TX, USA). Between-group heterogeneity was assessed using Cochran’s Q-test and the I 2 index. We conducted influence analysis by omitting each study to find potential outliers. Statistical analysis The exome sequence data were analysed with a χ 2 -test using PLINK software ( http://pngu.mgh.harvard.edu/~purcell/plink , version 1.07) and the parameter set ‘—assoc’. The OR and MAF of the affected and unaffected samples were calculated at the same time. The allelic and genotypic distributions between the different groups were compared using a χ 2 -test. For the low-frequency mutations (MAF <5%), SKAT-O was used. SKAT-O [36] is a SNP set-level (for example, a gene or a region) test for the association between a set of rare or common variants and dichotomous or quantitative phenotypes. SKAT aggregates individual score test statistics of SNPs in a SNP set and efficiently computes SNP set-level P values. A meta-analysis across cohorts was performed using Stata/SE version 11.0 (Stata Corp.). Accession codes: The sequence data from the patient samples have been deposited in [NCBI dbSNP] under the accession codes 1558270999, 1558271000–1558279999, 1558280000–1558289999 and 1558290000–1558293806. How to cite this article: Huang, L.-Z. et al. Whole-exome sequencing implicates UBE3D in age-related macular degeneration in East Asian populations. Nat. Commun. 6:6687 doi: 10.1038/ncomms7687 (2015).